The stimulus-evoked population response in visual cortex of awake monkey is a propagating wave Propagating waves occur in many excitable media and were recently found in neural systems from retina to neocortex. While propagating waves are clearly present under anaesthesia, whether they also appear during awake and conscious states remains unclear. One possibility is that these waves are systematically missed in trial-averaged data, due to variability. Here we present a method for detecting propagating waves in noisy multichannel recordings. Applying this method to single-trial voltage-sensitive dye imaging data, we show that the stimulus-evoked population response in primary visual cortex of the awake monkey propagates as a travelling wave, with consistent dynamics across trials. A network model suggests that this reliability is the hallmark of the horizontal fibre network of superficial cortical layers. Propagating waves with similar properties occur independently in secondary visual cortex, but maintain precise phase relations with the waves in primary visual cortex. These results show that, in response to a visual stimulus, propagating waves are systematically evoked in several visual areas, generating a consistent spatiotemporal frame for further neuronal interactions. Propagating waves of cortical activity have been a longstanding source of interest in neuroscience, from macroscopic scales spanning multiple cortical areas [1] to microscopic scales involving single neurons [2] . Since the recent introduction of multichannel recording techniques capable of resolving the dynamics of single cortical areas [3] , [4] , the spatiotemporal structure of activity in these mesoscopic cortical regions has become a prime subject of study. With these methods, stimulus-evoked propagating waves have been observed in several sensory cortices of the anaesthetised animal [5] , [6] , [7] , [8] , [9] , [10] , [11] , [12] , [13] , [14] . In awake preparations, however, the results are still unclear. In recent advances, multielectrode array recordings have uncovered travelling high-frequency gamma- and beta-band oscillations propagating across the primary visual [15] and motor [16] cortices of the monkey, and fast wave propagation in the auditory cortex of the awake cat [17] ; further, voltage-sensitive dye (VSD) imaging studies have observed propagating waves spanning large parts of the cerebral cortex in the awake rodent [18] , [19] , [20] . Nevertheless, the central question here still remains: does the stimulus-evoked population response in primary sensory cortex during waking states remain stationary at the point of thalamocortical input, or propagate across some extent of the cortical area? This question has serious implications for models of cortical coding [21] . While VSD imaging in the awake monkey is an ideal method to provide an answer, with its inherently high spatial and temporal resolution [22] , the first VSD imaging studies in the primary visual cortex have reported a spread of activity in the stimulus-evoked population response not clearly consistent with a stationary pulse or propagating wave [23] , [24] , [25] , [26] . The results of these first studies in the awake monkey were based on trial-averaged data, however, and given the well-known sensitivity of propagating waves in vivo to trial averaging [10] , [27] , it is possible that propagating waves on the single-trial level were attenuated by the averaging procedure. Here, to rigorously quantify the spatiotemporal dynamics underlying the population response in the awake monkey, we designed a phase-based method that works on unsmoothed data at the single-trial level, and provides a quantitative means to detect propagating waves in noisy multichannel data. We used data denoised for single-trial analysis [28] , and sought to distinguish unambiguously between a stationary population response (termed here a ‘Gaussian pulse’) and a spatiotemporally structured propagating wave. With this methods, we demonstrate that the stimulus-evoked population response is a propagating wave that travels across a large section of visual cortex in the awake monkey. On no-stimulus ‘blank’ trials, intermittent spontaneous propagations also occur. The evoked propagation occurs during all tested visual stimulation paradigms, and shows an intrinsic reliability: while wave onset is variable across trials, the phase variability of the waves does not increase during their course across cortical space, indicating a propagation substrate with a highly consistent propagation speed. The simplest mechanism accounting for this is the horizontal fibre network of the superficial cortical layers; using a topographic spiking network model, we confirm horizontal fibres can mediate such reliability under very general conditions. A direct consequence of this observation is that if two cortical areas are activated by a visual stimulus with short latency difference (such as primary and secondary visual cortex), then the propagations induced in these areas should be correlated in their course across cortical space. Indeed, we observe a significant correlation of stimulus-evoked waves in those two areas. Such a consistent spatiotemporal organization across neocortical circuits may be an important feature of the network-level computations in visual cortex during awake, ‘activated’ cortical states. VSD Imaging on the Single-Trial and Trial-Averaged Level For the experiments analysed in this study, the primary and secondary visual areas (V1 and V2) of the macaque monkey were imaged under spontaneous and stimulus-evoked conditions. The recording chamber was positioned over an area spanning portions of these cortical areas (18 mm diameter, Fig. 1a ; see Methods). Stimulation with a short (50 ms), small Gaussian blob evoked a fast response, which peaked within 50–100 ms after stimulus onset ( Fig. 1b , mean±s.d.). Noting the temporal characteristics, we selected a frequency band encompassing this fast response (5–20 Hz) for all further analysis. 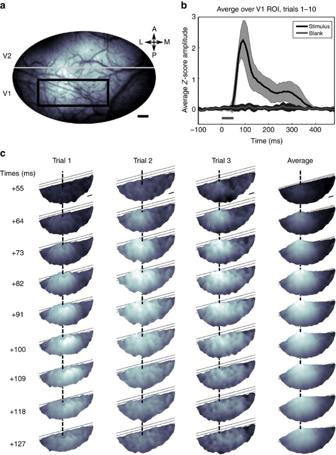Figure 1: Imaged cortical area and stimulus response time course. (a) Vasculature pattern. Black rectangle indicates V1 ROI for response inFigs 3,4. Black bars indicate 1 mm spatial scale throughout this work (here, bottom right). (b) Average time course in the V1 ROI for stimulus (black) and blank (grey) conditions, averaged over first 10 trials (mean±s.d.). The grey bar from 0–50 ms marks stimulus presentation. (c) Surface plots of the response, for three single trials and the trial average. Individual frames are smoothed with a Gaussian (0.23 mm s.d.), and scaled to the maximumZ-score in the trial. Horizontal black lines indicateZ-scores of 0, 1 and 2. Dashed vertical lines provide a visual reference across surface plots. Figure 1: Imaged cortical area and stimulus response time course. ( a ) Vasculature pattern. Black rectangle indicates V1 ROI for response in Figs 3 , 4 . Black bars indicate 1 mm spatial scale throughout this work (here, bottom right). ( b ) Average time course in the V1 ROI for stimulus (black) and blank (grey) conditions, averaged over first 10 trials (mean±s.d.). The grey bar from 0–50 ms marks stimulus presentation. ( c ) Surface plots of the response, for three single trials and the trial average. Individual frames are smoothed with a Gaussian (0.23 mm s.d. ), and scaled to the maximum Z -score in the trial. Horizontal black lines indicate Z -scores of 0, 1 and 2. Dashed vertical lines provide a visual reference across surface plots. Full size image Figure 1c illustrates the difference between the single-trial and trial-averaged level in these data. Smoothed surface plots of the stimulus-evoked VSD responses in three trials are plotted alongside the trial-averaged data (animations available online as Supplementary Movies 1–4 ). The form of the response is clearly different between the single-trial and trial-averaged data. A detailed inspection of the surface plots on the single-trial level shows that activity first emerges proximally (near the vertical reference line) and is followed in later frames by the development of stronger activity at more distal locations, suggesting the presence of a propagating wave. In contrast, on the trial-averaged level, distal responses are heavily attenuated as a result of the averaging, resulting in a spatiotemporal pattern similar to a Gaussian pulse (see Introduction). Nevertheless, while propagations seem to be present on the single-trial level, the phase relationship between proximal and distal sites cannot be clearly established in these amplitude-domain, smoothed surface plots, where the detailed spatiotemporal dynamics remain obscured. For this reason, we need more sophisticated methods to characterize the ‘phase latency’ of individual channels in the unsmoothed data. Phase latency method To quantify the spatiotemporal properties of visual responses, we compute instantaneous phase at each pixel via the analytic signal framework [16] , [29] , [30] , wherein a real-valued, narrowband time series on channel can be written as a complex exponential: where H denotes the Hilbert transform, the instantaneous amplitude of channel i at time t , denotes the instantaneous phase of the same, and j is the imaginary unit. To illustrate this concept, Fig. 2a depicts the representation of a damped oscillation in the real, imaginary and complex planes via the analytic signal, in order to provide an example of the transformation of a real signal into a complex phasor. 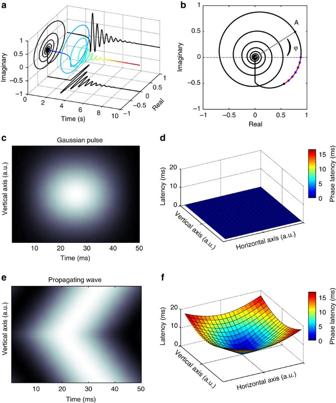Figure 2: Phase latency method. (a) The real, imaginary, and complex plane projections of the analytic signal (coloured by heat in time) for a damped oscillation make explicit the decomposition of a real signal into a complex phasor30. (b) The complex plane projection in (a) is used in this work to analyse instantaneous amplitude (A, complex modulus) and phase (φ, complex angle) in the real signal. The red curve in (b) illustrates the interval over which an example phase latency calculation takes place. (c) A vertical section through time of a representative Gaussian pulse. Note the spatial axes have arbitrary units (a.u.). (d) Phase-latency map for the Gaussian pulse response depicted in (c). Note that the minimum latency has been subtracted from all maps, to aid visualization. (e) A section through time of a representative target wave. (f) The phase-latency map for this example captures the spatiotemporal organization in these data. Figure 2: Phase latency method. ( a ) The real, imaginary, and complex plane projections of the analytic signal (coloured by heat in time) for a damped oscillation make explicit the decomposition of a real signal into a complex phasor [30] . ( b ) The complex plane projection in ( a ) is used in this work to analyse instantaneous amplitude ( A , complex modulus) and phase ( φ , complex angle) in the real signal. The red curve in ( b ) illustrates the interval over which an example phase latency calculation takes place. ( c ) A vertical section through time of a representative Gaussian pulse. Note the spatial axes have arbitrary units (a.u.). ( d ) Phase-latency map for the Gaussian pulse response depicted in ( c ). Note that the minimum latency has been subtracted from all maps, to aid visualization. ( e ) A section through time of a representative target wave. ( f ) The phase-latency map for this example captures the spatiotemporal organization in these data. Full size image In this work, we specifically consider the latency in absolute time to a given phase crossing as the phasor at each channel rotates in the complex plane (‘phase latency’, Fig. 2b ). The calculation of phase latency starts from a selected point in the time series (first black point, Fig. 2b ), and consists of finding the two samples on either side of a given phase crossing (2 π throughout). Linear interpolation based on the instantaneous frequency of the signal between these two points returns the exact time for the crossing within the interval. This calculation is made independently for all channels in the bandpass-filtered, spatially unsmoothed data. By analysing spatial patterns in the phase latency across channels, we can unambiguously distinguish between stationary pulses and propagating waves in VSD imaging data. To clarify this distinction, we focused on two idealized models for the form of the population response: a spatiotemporally separable, stationary ‘Gaussian pulse’ and a spatiotemporally inseparable propagating wave. Note that here we use ‘pulse’ as a purely temporal concept, indicating a lack of phase organization across space, whereas a ‘propagating wave’ indicates this spatiotemporal organization, for both single- and multi-cycle events. We write the Gaussian pulse as a separable function of space and time: where g(x) represents a Gaussian profile in space and h ( t ) is a sinusoidal response time course , with amplitude A , spatial spread σ , and angular frequency ω , over one cycle of response. Given this definition of the Gaussian pulse, its analytic signal representation z ( x , t ) becomes: which has the properties discussed above—phasors rotating in the complex plane, each with identical phase angle, whose amplitudes are modulated by a Gaussian in space (see Methods—Analytic Signal Representation of the Gaussian Pulse). Clearly, because of the spatiotemporal separability of this model, the phase-latency map calculated for a representative Gaussian pulse is flat, exhibiting no organization across space ( Fig. 2c,d ). By contrast, the phase-latency map calculated for an expanding target wave (sin( λr − ωt ), where r is the norm of the distance vector from the source) captures the phase offset across space, producing a basin centred on the wave source ( Fig. 2e,f ). It is important to emphasize that, in contrast, a latency analysis in the amplitude domain cannot distinguish between Gaussian pulses and propagating waves ( Supplementary Fig. 1 ). Several tests were made with various signals and sources of noise to ensure that the phase latency method is robust against false-positive propagation detections ( Supplementary Fig. 2 ). Phase-latency maps reveal spontaneous and evoked waves Phase-latency maps were calculated pixel by pixel starting from +72.7 ms after stimulus onset, then smoothed for purposes of visualization (Methods). Individual phase-latency maps at the single-trial level show a clear increase in latency with distance from the source of the basin ( Fig. 3a ), in the range expected for a propagation mediated by the horizontal fibre network [6] , [31] , [32] . While no spatiotemporal organization was observed in the blank trial data at the corresponding temporal point, we did observe several instances of spontaneous propagating waves, with similar propagation speed as the evoked, emerging at various spatial and temporal points during the no-stimulus imaging sessions ( Fig. 3b ). Note that the size, but not the position, of the ROI in Fig. 3b corresponds to that in Fig. 3a . 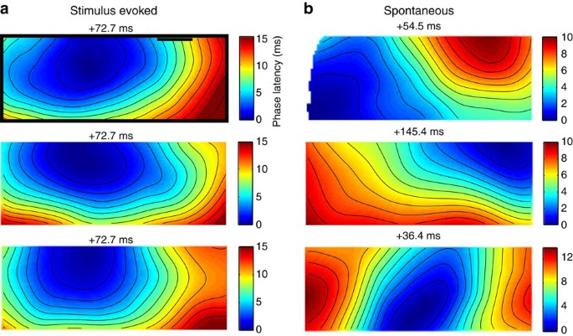Figure 3: Single-trial evoked and spontaneous waves in awake monkey. (a) Single-trial phase-latency maps for V1 ROI in the 50 ms stimulus presentation condition, from trials 1, 3 and 10. These maps are calculated at +72.7 ms after stimulus onset. Note black box in top panel corresponds to V1 ROI inFig. 1a. (b) Phase-latency maps for spontaneous waves observed during no-stimulus, blank conditions. Note the varying colour axis and temporal points for the spontaneous maps. Figure 3: Single-trial evoked and spontaneous waves in awake monkey. ( a ) Single-trial phase-latency maps for V1 ROI in the 50 ms stimulus presentation condition, from trials 1, 3 and 10. These maps are calculated at +72.7 ms after stimulus onset. Note black box in top panel corresponds to V1 ROI in Fig. 1a . ( b ) Phase-latency maps for spontaneous waves observed during no-stimulus, blank conditions. Note the varying colour axis and temporal points for the spontaneous maps. Full size image We next addressed whether these propagations occurred consistently across trials. For this, individual phase-latency maps were calculated at the same temporal point for trials 1–10, smoothed and then averaged. This average phase-latency map ( Fig. 4a , top) again shows a clear increase in latency with distance from the source, consistent with the single-trial maps. No spatiotemporal organization is observed in the blank trial data at the corresponding temporal point, which produces a flat phase-latency map ( Fig. 4a , bottom). This trial-average over phase-latency maps is much less sensitive to noise than the trial-average over the signal, first because the waves are extracted in the individual trials before the average, and second because this measure is insensitive to amplitude fluctuations ( cf. Fig. 1c ). 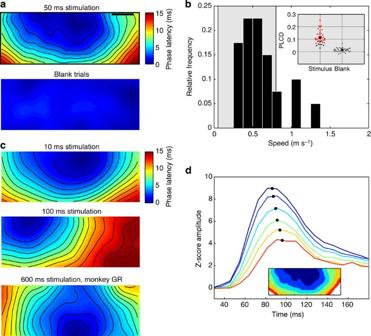Figure 4: Stimulus-evoked propagating waves in V1 of the awake monkey. (a) Average phase-latency map for V1 ROI for stimulus (top) and blank (bottom) data. (b) Propagation speeds extracted from the slope of the phase latency with distance in the unsmoothed maps, 50 ms stimulus presentation condition. (Shaded area) biophysically plausible range of horizontal conduction speeds (0.05–0.8 m s−1). (Inset) phase latency correlation with distance (PLCD), stimulus (black) and blank (grey) conditions. Trials with positive detections are marked in red. Mean correlation coefficient±s.e.m. plotted with larger black dots (Fisherz-transform). Note that error bars are obscured behind the dots. (c) Additional phase-latency maps across stimulus presentation length (10 and 100 ms, top and middle), and across animals (600-ms stimulus, monkey GR). Note only significant trials are included in this representation. Stimulus coordinates were 3.5°, 3° and 5° below the horizontal meridian, respectively, and 3° left of the vertical in the 600 ms condition. (d) ROIs of increasing phase latency (bottom inset, concentric regions coded by heat) show a temporal offset with distance (time courses, matching colour code). Interpolated maxima plotted directly on time courses (black dots). Figure 4: Stimulus-evoked propagating waves in V1 of the awake monkey. ( a ) Average phase-latency map for V1 ROI for stimulus (top) and blank (bottom) data. ( b ) Propagation speeds extracted from the slope of the phase latency with distance in the unsmoothed maps, 50 ms stimulus presentation condition. (Shaded area) biophysically plausible range of horizontal conduction speeds (0.05–0.8 m s −1 ). (Inset) phase latency correlation with distance (PLCD), stimulus (black) and blank (grey) conditions. Trials with positive detections are marked in red. Mean correlation coefficient±s.e.m. plotted with larger black dots (Fisher z -transform). Note that error bars are obscured behind the dots. ( c ) Additional phase-latency maps across stimulus presentation length (10 and 100 ms, top and middle), and across animals (600-ms stimulus, monkey GR). Note only significant trials are included in this representation. Stimulus coordinates were 3.5°, 3° and 5° below the horizontal meridian, respectively, and 3° left of the vertical in the 600 ms condition. ( d ) ROIs of increasing phase latency (bottom inset, concentric regions coded by heat) show a temporal offset with distance (time courses, matching colour code). Interpolated maxima plotted directly on time courses (black dots). Full size image Nevertheless, these smoothed phase-latency maps do not provide a quantitative criterion for the distinction between a significant propagation and background noise; for this, we use the original, unsmoothed phase-latency maps to test for a linear relationship between phase latency and distance (Methods). We extracted the propagation speed from the slope of this relationship across 40 trials in the 50-ms stimulus presentation condition ( Fig. 4b ). Propagation speeds followed a positively skewed distribution, ranging from 0.25–1.35 m s −1 , with a median speed of 0.57 m s −1 and a median absolute deviation of 0.18 m s −1 , in close correspondence to the observed range of horizontal conduction speeds in monkey V1 (ref. 32 ). The correlation coefficient ( ρ d ) for stimulus (black points) and blank (grey points) conditions is given in the inset. Positive detection of a propagating wave for each trial at the given time point was determined by significance of the correlation coefficient ( α =0.01, one-tailed t -test, H 0 : ρ d =0, H 1 : ρ d >0, with Bonferroni correction), coupled with a criterion for the propagation speed determined from the slope of the regressor line to be within the biophysically plausible range of horizontal conduction speeds (0.05–0.8 m s −1 , shaded area in Fig. 4b ) [6] , [31] , [32] . Under these dual detection criteria, we found stimulus-evoked propagations over the imaging array in 32 of 40 trials (80.0% detection rate, red points in Fig. 4b , inset). In contrast, for the blank trial data, no propagations were detected at the chosen temporal point. We analysed additional stimulus presentation conditions in two animals ( Fig. 4c , 10- and 100-ms stimulus in monkey WA, and 600-ms stimulus in monkey GR). The phase-latency maps for each condition (also calculated at +72.7 ms) contained similar modulations across space for the 10-, 100- and 600-ms stimuli (80.0, 52.6 and 20% detection rate, respectively). No major differences were observed in the features of the waves between animals and stimulus presentation durations; rather, whether waves could be detected on the single-trial level was related to the signal–to-noise ratio achieved during the individual imaging session. Note that shifts of phase latency minima reflect different visuospatial coordinates for stimuli in each condition, and were verified to correspond to the expected point of thalamocortical input. As previously, no propagations were detected in the matched blank trial data. As a control on the results derived from the phase latency method, we divided the V1 ROI into successive regions by their measured phase latency (six regions total in the smoothed maps, in 2-ms bins), and averaged all channels across trials and within the region in the unfiltered data from the 50-ms stimulus presentation condition ( Fig. 4d ). Despite the fact that the process of trial-averaging dramatically attenuates the spatiotemporal frequency components observed on the single-trial level ( cf. Fig. 1 ), by averaging over trials and region defined by phase latency calculated in the bandpass data, we are able to recover a trial-consistent phase offset even in the unprocessed data ( Fig. 4d , black dots). This control analysis confirms that the propagating response is well characterized by the phase information in the 5–20 Hz frequency band, and rules out artifacts in the phase representation or bandpass filtering of the data. Further, it is important to note that additional checks confirmed the 5–20 Hz frequency band chosen here captures the full waveform of the fast stimulus-evoked population response well: as an example, repeating the analysis in Fig. 4b with a lowpass filter at 27.5 Hz (that is, the lower half of the available frequency spectrum) results in a similar number of wave detections (34 of 40 trials in the 50-ms stimulus condition), while a highpass filter at 27.5 Hz results in zero wave detections. Phase gradient Having confirmed the existence of stimulus-evoked propagating waves of activity in these VSD imaging data, we then examined the response wavevectors taken from the spatial gradient of phase at each time point. 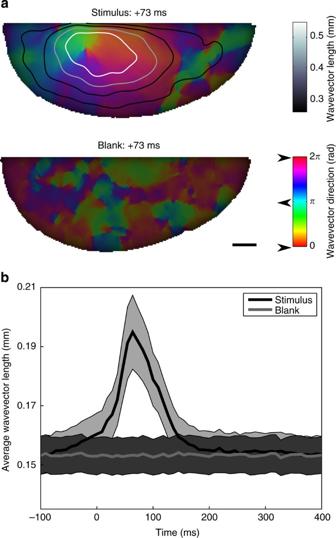Figure 5: Phase gradient magnitude and direction plot. (a) Wavevector plot of the phase gradient in the stimulus (top) and blank trials (bottom), averaged over the first 10 trials of the 50-ms stimulus condition. Propagation direction is represented by pixel hue (colour bar, bottom right), with wavevector length represented by pixel luminance and grayscale contours (colour bar, top right). (b) Phase gradient averaged over V1 ROI, for the stimulus (black) and blank (grey) conditions, mean±s.e.m. Following previous work [16] , [33] , [34] , the wavevector at time t is: Figure 5a depicts the phase gradient at +72.7 ms, averaged over the first ten trials of the session for the stimulus (top) and blank (bottom) conditions. In this wavevector plot over all V1 channels, a ‘pinwheel’ of colour hues in a region of high phase gradient magnitude marks the source of propagation during the response epoch ( Fig. 5a , top). In contrast, the wavevector plot for the blank trial data has low-phase gradient magnitude and no such spatial organization ( Fig. 5a , bottom). To estimate the spatial extent of the propagations in these data, we calculated the contour at 2.32 standard deviation (s.d.) values away from the mean of the phase gradient magnitude in the blank trial data (attained by <1% of values in the blank), and delimited a contiguous, approximately elliptical region on the wavevector map in the stimulus condition, with a long axis of 7.5 mm and a short axis of 3.7 mm (calculated via normalized second central moments of the equivalent ellipse), compatible with known anatomy [35] , [36] and reported spatial spread [23] , [26] . Using a magnification factor of 0.35° mm −1 at an eccentricity of 3.5° (refs 37 , 38 ) and an anisotropy index of 1.5 along the inferior vertical meridian [39] , this cortical area corresponds to an ellipse of 2° on the horizontal axis and 2.7° on the vertical axis of the visual field. In looking at the phase gradient wavevector length time series averaged over the V1 ROI for the first 10 trials (mean±s.e.m., Fig. 5b ), a sharp phasic increase occurs during the stimulus response epoch, in comparison with the phase gradient time course from the blank trial data (here, high pass filtered with 5 Hz cutoff frequency). These additional measurements based on the spatial gradient of phase clarify the spatial extent of the propagations observed in the data, and corroborate their appearance in a consistent manner across trials. Figure 5: Phase gradient magnitude and direction plot. ( a ) Wavevector plot of the phase gradient in the stimulus (top) and blank trials (bottom), averaged over the first 10 trials of the 50-ms stimulus condition. Propagation direction is represented by pixel hue (colour bar, bottom right), with wavevector length represented by pixel luminance and grayscale contours (colour bar, top right). ( b ) Phase gradient averaged over V1 ROI, for the stimulus (black) and blank (grey) conditions, mean±s.e.m. Full size image Trial variability and network model We next analysed the variability of these propagations in time. During an oscillatory epoch, the phase distribution over channels will in general be peaked and have a well-defined mean direction (MD) [40] . The distribution of MDs (+64 ms, 5–20 Hz frequency band) across 40 trials spans more than a quarter-cycle in the 50-ms stimulus condition ( Fig. 6a , black arrows); given the mean instantaneous frequency at this temporal point (11.26 Hz), this span implies a variability on the order of tens of milliseconds (29.08 ms). Note that these results were verified at several time points throughout the stimulus response. 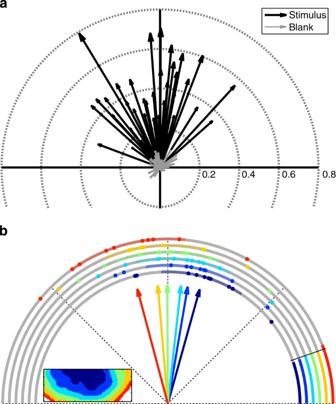Figure 6: Variability analysis. (a) Mean direction of phase distribution at +64 ms, scaled by length of the resultant vector, for 50-ms stimulus (black arrows) and blank (grey) conditions. (b) Mean direction across individual phase-latency regions (inset at bottom left, as defined inFig. 4d), first 10 trials of the stimulus condition (coloured points). (Coloured arrows) mean direction of the cross-trial distribution. (Shaded regions) mean direction±angular deviation. (Coloured regions, bottom right) angular deviations, with line through mean of the deviations for visualization (black line). Figure 6: Variability analysis. ( a ) Mean direction of phase distribution at +64 ms, scaled by length of the resultant vector, for 50-ms stimulus (black arrows) and blank (grey) conditions. ( b ) Mean direction across individual phase-latency regions (inset at bottom left, as defined in Fig. 4d ), first 10 trials of the stimulus condition (coloured points). (Coloured arrows) mean direction of the cross-trial distribution. (Shaded regions) mean direction±angular deviation. (Coloured regions, bottom right) angular deviations, with line through mean of the deviations for visualization (black line). Full size image By dividing this analysis over-phase latency regions (as in Fig. 4d ), we studied this variability across space ( Fig. 6b ). Interestingly, while the mean directions of the cross-trial MD distribution in each region experience a 30.4-degree phase shift across space (reflecting the underlying propagating wave dynamics), the angular deviations differ by no more than 2.5 degrees ( Fig. 6b , lower right). In other words, the cross-trial phase variability of the waves does not increase with distance from their source. This strongly suggests that the intrinsic dynamics of the propagations are invariant across trials and space, and that the observed trial variability in these propagations can be explained by simple temporal shifts of the propagating wave from trial to trial. To investigate possible mechanisms explaining these observations, we studied a one-dimensional topographic spiking network model composed of excitatory and inhibitory neurons operating in a balanced regime, with local connections and linear conduction delays (Methods), and with length L (7.0 mm, matched to the spatial extent of the wave propagation, see Results–Phase Gradient). Stimulation of the middle 100 excitatory cells in the network with a Gaussian spike packet (centre time μ sp ; Fig. 7a ) ignites a wave of subthreshold activity, which propagates along a rigid spatiotemporal path, determined by the fixed axonal conduction delays and rise time of the postsynaptic potential ( Fig. 7b ). We divided the network into six regions based on distance from the stimulation zone (coloured regions; Fig. 7a,b ) and used the analytic signal representation for the response waveform, as with the experimental data (Methods). 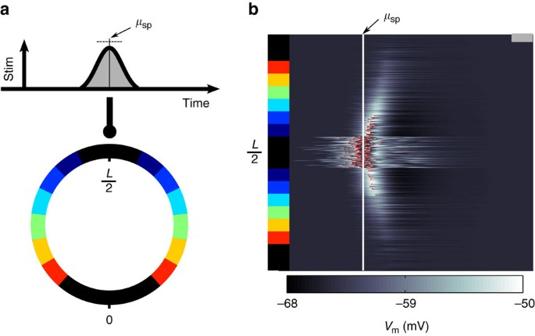Figure 7: A spiking network model of the trial-invariant response. (a) Schematic of the network model and stimulation paradigm. The network is composed of excitatory and inhibitory cells operating in a balanced regime, and is wrapped onto a one-dimensional ring of lengthLwith distance-dependent connections. A Gaussian spike packet is delivered to the network with a centre timeμsp. Six regions with increasing distance from the edge of the stimulation zone are selected for analysis of their averaged response waveform. (b) Example of a stimulus giving rise to a wave of activity. The membrane potential (Vm) across all cells in the excitatory population is plotted in grayscale, with analysis regions depicted at left. Spikes are depicted on the membrane potential time courses by red dots. Figure 7: A spiking network model of the trial-invariant response. ( a ) Schematic of the network model and stimulation paradigm. The network is composed of excitatory and inhibitory cells operating in a balanced regime, and is wrapped onto a one-dimensional ring of length L with distance-dependent connections. A Gaussian spike packet is delivered to the network with a centre time μ sp . Six regions with increasing distance from the edge of the stimulation zone are selected for analysis of their averaged response waveform. ( b ) Example of a stimulus giving rise to a wave of activity. The membrane potential ( V m ) across all cells in the excitatory population is plotted in grayscale, with analysis regions depicted at left. Spikes are depicted on the membrane potential time courses by red dots. Full size image The most likely mechanism underlying the trial-invariant dynamics observed in our experiments is a predominantly monosynaptic propagation carried by the horizontal fibre network of the superficial cortical layers, whose axonal conduction velocities are solely a function of the axonal diameter [41] , and are therefore fixed from trial to trial. We used this spiking network model to further understand how this mechanism could produce the phase distributions observed experimentally in two ways: by adding variability in the timing of the input to the system, or by adding variability in the axonal conduction velocity. The rationale for the choice in parameters studied is this: in observing the constant phase variability across distance (as in Fig. 6b ), we postulate that this is due to a static underlying mechanism, observed under various sources of noise. If this were not the case, however, and the spatiotemporal dynamics observed in our analysis were mediated by some other process, such as a gain-control mechanism [25] , we would expect variability in the apparent conduction speed, as well, which would then manifest as an increase in angular deviation with distance. To study these two sources of variability, the stimulation paradigm is repeated over ten trials, and the cross-trial phase distribution is plotted as in Fig. 6b . With no additional source of variability in the system, all cross-trial phase distributions have zero angular deviation, as the response phase is totally consistent from trial to trial ( Fig. 8a ). If the centre time of the Gaussian spike packet (μ sp ) is drawn from a uniform distribution ranging from 95 to 105 ms, the angular deviations become nonzero, but remain constant across analysis regions (input jitter; Fig. 8b ), as in the experimental data. If the axonal conduction speed for the network in each trial is drawn from a uniform distribution (from 0.2–0.5 ms −1 ), however, the angular deviations then increase markedly with distance from the source (speed variability; Fig. 8c ), in stark contrast to the experimental data. The rate of the increase in angular deviation with distance from the stimulation zone is directly proportional to the range of the uniform distribution from which the axonal conduction speed for the network is drawn at each trial ( Fig. 8d , lines of increasing brightness). Note that additional control simulations were performed to test that the combination of these two sources of variability, rather than being mutually obscuring, produces an even larger increase in variability with distance than either source in isolation. 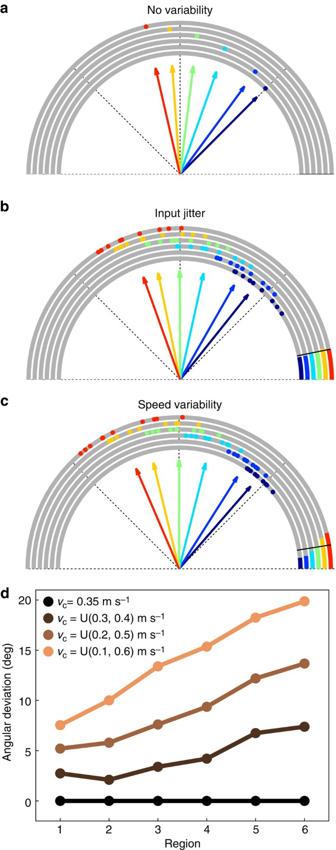Figure 8: Input jitter explains the observed phase distribution, while speed variability does not. (a) Cross-trial phase distribution over analysis regions, plotted as inFig. 6b, over 10 iterations. The cross-trial phase distributions have zero angular deviation, as no variability is present in the system. (b) Cross-trial phase distribution under 10-ms jitter in the centre time of the Gaussian spike packet input. The angular deviation remains constant across analysis regions. (c) Phase distribution under speed variability (uniform distribution ranging from 0.2 to 0.5 m s−1). The angular deviation increases markedly across analysis regions. (d) The angular deviation across regions is plotted for several uniform distributions ofεc, with a range expanding around the centre speed 0.35 m s−1. Figure 8: Input jitter explains the observed phase distribution, while speed variability does not. ( a ) Cross-trial phase distribution over analysis regions, plotted as in Fig. 6b , over 10 iterations. The cross-trial phase distributions have zero angular deviation, as no variability is present in the system. ( b ) Cross-trial phase distribution under 10-ms jitter in the centre time of the Gaussian spike packet input. The angular deviation remains constant across analysis regions. ( c ) Phase distribution under speed variability (uniform distribution ranging from 0.2 to 0.5 m s −1 ). The angular deviation increases markedly across analysis regions. ( d ) The angular deviation across regions is plotted for several uniform distributions of ε c , with a range expanding around the centre speed 0.35 m s −1 . Full size image This network model reproduces the cross-trial phase distributions observed in the experimental data under very general conditions. Moreover, the simplicity of the mechanism studied does not preclude its uniqueness: other mechanisms, whose apparent conduction speeds are affected by the ongoing dynamics in the network, do not show this non-increase in phase variability across space. In this way, we demonstrate not only that the propagation must be mediated by the horizontal fibre network of the superficial cortical layers, but also that this mechanism of propagation generation provides a unique physical substrate for delivering a precisely timed event with trial-invariant dynamics (e.g. under temporal variability in the input), preserving across trials temporal patterns in the population response over several millimetres of primary visual cortex. Dual, independent propagations in V1 and V2 The horizontal propagation mechanism furthermore directly implies that propagations in V1 and V2 should be synchronized in their course across cortical space, as these areas are retinotopically activated by a visual stimulus in a fixed, rapid temporal sequence [42] , [43] . Specifically, because these areas are activated with comparable response latencies (points labelled A in Fig. 9a ) and the horizontal fibre network in each area will carry the propagations with similar speeds, the propagations should reach points in the cortex with similar distance from the source at the same time (points labelled B in Fig. 9a ). In accordance with this expectation, we did in fact observe dual stimulus-evoked propagating waves travelling across V1 and V2, respectively ( Fig. 9b ). Next, to verify that the propagations observed in this region are also likely mediated by the horizontal fibre network, we performed the trial variability analysis in V2, just as in Fig. 6b , and indeed observed that the cross-trial phase variability similarly does not increase with distance ( Fig. 9c ). 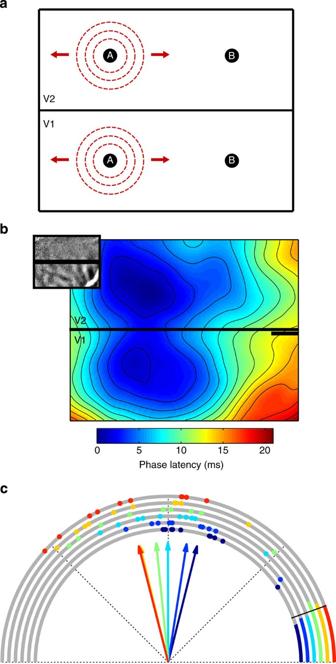Figure 9: Dual propagating waves in V1 and V2. (a) Schematic of dual stimulus-evoked propagations in V1 and V2. Simultaneous input atAevokes a propagating wave. Because the waves are carried by horizontal fibres (with nearly constant propagation velocity), the propagations will arrive in a synchronized fashion atB. (b) Phase-latency map at V1/V2 border, 50-ms stimulus condition, average over 10 trials. (Inset) ocular dominance map. (c) Cross-trial phase distribution calculated over analysis regions, as inFig. 6b. Figure 9: Dual propagating waves in V1 and V2. ( a ) Schematic of dual stimulus-evoked propagations in V1 and V2. Simultaneous input at A evokes a propagating wave. Because the waves are carried by horizontal fibres (with nearly constant propagation velocity), the propagations will arrive in a synchronized fashion at B . ( b ) Phase-latency map at V1/V2 border, 50-ms stimulus condition, average over 10 trials. (Inset) ocular dominance map. ( c ) Cross-trial phase distribution calculated over analysis regions, as in Fig. 6b . Full size image To summarize the situation observed here, our results suggest that the retinotopic feedforward stream rapidly activates primary and secondary visual cortex in succession, generating two independent waves propagating along the horizontal network in each area. These two waves, which both express consistent dynamics indicative of the horizontal network ( Figs 6b and 9c ) and similar spatiotemporal dyamics ( Figs 4a,c and 9b ), are thus expected to exhibit phase correlations across time for each pair of pixels in individual trials. Interestingly, because of the smooth retinotopic organization in V1 and V2, this correlation across cortical space will also correspond to correlation in retinotopic space. To quantify this effect systematically, we considered spatial sections of V1 and V2, aligned by flipping V2 vertically across the border, and computed the circular correlation coefficient ( ρ cc ) of the instantaneous phase between each pair of aligned pixels at each point in time ( Fig. 10a ; see Methods). Note that this calculation is performed in the temporally filtered but spatially unsmoothed data, to preclude any smoothing artifact from introducing spurious correlation. In the average over the first ten trials of the 50-ms stimulus presentation condition, a sharp, transient increase in the correlation coefficient between V1 and V2 is evident (black line, mean±s.e.m., Fig. 10a ), indicating that a similar pattern of phase develops in each cortical area during the wave propagation epoch. No such transient increases in the interarea correlation coefficient were observed during the matched blank trials (dark grey, Fig. 10a ). Interestingly, shuffling the spatial position of each time course in the imaging array removes this transient correlation (light grey, Fig. 10a ), indicating that it is indeed due to specific spatial patterns shared between the two areas. Even more interestingly, when only the subset of time courses corresponding to the points nearest the thalamocortical input is shuffled (light blue, dashed, Fig. 10a ), the transient increase remains nearly unchanged from the stimulus case, indicating that the spatial pattern of the phase responsible for this transient increase is diffuse, spread through a large extent of the individual cortical regions. Such diffuse, correlated phase patterns indicate a novel large-scale organization of the dynamics in these first two regions of the visual hierarchy, which presumably extends to areas higher in the visual hierarchy, and which could serve to organize computations in the visual system across space and time. 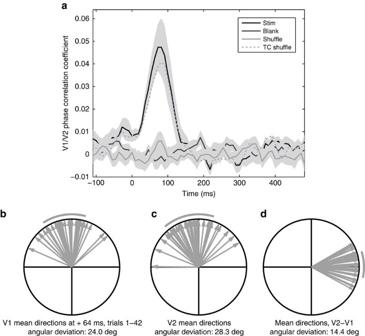Figure 10: Propagating waves in V1 and V2 are correlated but independent. (a) Interarea phase correlations, mean±s.e.m. for stimulus (black), blank (dark grey), shuffled stimulus (light grey) and thalmocortical input control (dashed light blue) cases. (b) Mean direction distribution in V1 at +64 ms for the 50 ms stimulus condition. (Grey curve) angular deviation of the cross-trial MD distribution. (c) V2 MD distribution and angular deviation. (d) The angular difference of the MD distributions in V1 and V2 exhibits an angular deviation that is moderately decreased, but non-vanishing. Figure 10: Propagating waves in V1 and V2 are correlated but independent. ( a ) Interarea phase correlations, mean±s.e.m. for stimulus (black), blank (dark grey), shuffled stimulus (light grey) and thalmocortical input control (dashed light blue) cases. ( b ) Mean direction distribution in V1 at +64 ms for the 50 ms stimulus condition. (Grey curve) angular deviation of the cross-trial MD distribution. ( c ) V2 MD distribution and angular deviation. ( d ) The angular difference of the MD distributions in V1 and V2 exhibits an angular deviation that is moderately decreased, but non-vanishing. Full size image In light of this result, it is natural to ask further whether these dual, correlated waves in neighbouring cortical regions are in fact independent, or part of one continuous wave. To answer this question, we analysed to what extent the variability in the mean direction of the phase distribution in V2 is explained by the variability in V1 across trials by taking the circular difference of the MDs in each area ( Fig. 10b–d ). Both MD distributions in V1 and V2 have similar angular deviations (24.0 and 28.3 degrees, respectively), and similar phase values overall, leading to a distribution of the circular differences centred at zero radians ( Fig. 10d ), illustrating again the synchrony of these dual waves. Importantly, however, the angular deviation of this distribution of the differences between MDs is only moderately decreased relative to the angular deviation of the individual MD distributions in V1 and V2. This indicates that while part of the variability in V2 is explained by that of V1, the waves are not perfectly correlated, consistent with the interpretation that each wave is generated independently by the retinotopic feedforward volley, and then mediated by the horizontal fibre network of each cortical area in a predominantly monosynaptic fashion. Finally, it is important to specify that throughout this analysis, we did not observe a phase resetting, or second oscillation cycle, that would indicate the presence of a wave from either region crossing the border between the two. Thus, the propagating waves observed in both cortical areas imaged here seem to respect an anatomical border, in contrast to the wave dynamics observed in the visual cortex of the anaesthetised rat [10] . Whether this difference is due to variation among species or to cortical state will be an interesting topic for future research. While the existence of spontaneous and stimulus-evoked propagating waves during waking states in primary sensory cortices has been highly debated in recent years (see Sato et al . [44] ; Muller and Destexhe [45] for review), our analysis shows for the first time that these waves occur systematically in the awake, behaving monkey, and that these waves are consistently evoked on the great majority of trials. Furthermore, by analysing the temporal variability in these propagations across trials, we observe that the intrinsic neocortical dynamics are invariant apart from a variable onset time for each propagation. Using a network model, we confirm that the most likely propagation mechanism—a predominantly monosynaptic propagation mediated by the horizontal fibre network of the superficial cortical layers—produces trial-invariant dynamics as observed in the experimental data. In addition, we also find that the retinotopic feedforward stream, which activates primary and secondary visual cortex in rapid succession [42] , [43] , with short, fixed latency differences [46] , evokes a wave in V2 which then propagates nearly simultaneously with the wave in V1. These dual propagating waves induce in the two cortical areas correlated spatial patterns of phase, which establish a consistent spatiotemporal frame for further neuronal interactions, possibly including those in regions downstream in the visual hierarchy. Previous VSD imaging studies in primate visual cortex worked primarily on the level of trial-averaged data [5] , [23] , [25] , [26] , where the transient dynamics of the single-trial VSD response are heavily attenuated (see Fig. 1 ), and either did not specifically study the spatiotemporal form of the population response [5] , [23] , or observed synchronous dynamics early in the response (attributed to a gain-control mechanism) [25] . Here, working always on the single-trial level, we observe a consistent offset across space throughout the response ( Fig. 4d ) and a trial-invariant dynamics indicative of a propagation mechanism that remains static from trial to trial ( Figs 6 , 7 , 8 ). Together, these results conclusively demonstrate that the fast component of the stimulus-evoked VSD response is indeed a propagating wave mediated by the horizontal fibre network of the superficial cortical layers. To observe and characterize propagating waves in a primary sensory cortex of the awake animal, we have introduced a phase-based method representing the first step towards automated, nonparametric identification of arbitrarily shaped propagating waves in noisy multichannel data. Similar approaches have either restricted detection possibilities to plane wave phenomena [16] , or used a template matching approach in the amplitude domain [47] , which precludes the generality of the method and hinders its robustness to noise. Furthermore, this method is able to capture the transient, trial-variable single-cycle propagations observed in these data, which is difficult with methods based on the phase of Fourier components [9] , or spike-triggered averaging [48] . It is not to be claimed, however, that this method offers a fully automated approach at this stage; for example, the results in this study were fully and meticulously checked by visual inspection. With a complete characterization of the method on well-controlled surrogate data, however, fully automated detection of propagations in noisy data could soon become possible. It is thought that the majority of the VSD signal is due to dendritic activity of superficial neurons, with minor contributions due to spiking activity and to deep layers [49] . The waves detected in the VSD signal in this study thus correspond to transient depolarization of excitatory and inhibitory neurons travelling across the cortex, carried primarily by the horizontal fibre network of the superficial cortical layers [35] , [36] . Such transient depolarizations will affect the processing of future stimuli at distant points in visual cortex [6] , [7] , [26] , as ascending input will combine with the travelling depolarization at a correctly timed interval, changing the spiking response. Furthermore, because neurons during waking, ‘activated’ cortical states sit a few millivolts below threshold [50] , [51] , [52] , operating in a fluctuation-driven regime [53] , [54] , [55] , it is reasonable to expect that such input fluctuations will transiently change the spiking probability in the local circuit. Such possibilities will be the subject of future experimental and theoretical work. Finally, note that the phase latency correlations with distance observed in these data are significant, but not overly strong (see Fig. 4b ). Whether this is due to the noise inherent in VSD imaging on the single-trial level, or to the noisy, asynchronous-irregular type background activity that is the hallmark of the awake state [51] , remains to be addressed in future imaging studies, with continually improved signal-to-noise ratios. The horizontal fibre network has previously been implicated in active computational roles [6] , [7] , [26] , [56] , [57] , [58] , [59] . By proving here that the population response in awake monkey V1 and V2 is indeed a propagating wave, we implicate the horizontal fibre network in a much more specific function. Previous work has discussed the possibility that waves propagating across cortical maps could label sensory inputs with a unique phase [21] , and in this work, we have provided a conclusive experimental demonstration of the plausibility for such a computational role. In particular, the discovery that independent propagating waves in V1 and V2 maintain precise phase relations shows that, at least for these two areas, this coordinated activity will influence, and perhaps actively participate in, cortical computations. In light of these results, we suggest that the existence of propagating waves in awake, conscious states expands the basic function of cortical maps, as these spatiotemporal dynamics will animate these maps with well-defined phase relations both within and across regions. Surgical preparation Experiments were conducted on two male rhesus monkeys ( macaca mulatta , aged 5 and 8 years old). The monkeys were chronically implanted with a head-holder and a recording chamber located above the cortical areas V1 and V2 of the right hemisphere. The dura was surgically removed over a surface corresponding to the recording aperture (18 mm diameter) and a silicon-made artificial dura was inserted under aseptic conditions. Before each recording session, the cortex was stained with the VSD RH-1691 (Optical Imaging). For this, the optical chamber was opened, the artificial dura removed and the cortical surface was cleaned under strictly sterile conditions [60] . The dye solution was prepared in artificial cerebrospinal fluid at a concentration of 0.2 mg ml −1 , and filtered through a 0.2-μm filter. The recording chamber was filled with this solution and closed for 3 h. The chamber was then rinsed thoroughly with filtered artificial cerebrospinal fluid to wash off any supernatant dye, the artificial dura was placed back in position and the chamber was filled with transparent agar before closing with a transparent cover. During the recordings, the cortex was illuminated at 630 nm to excite the dye for 600–1,000 ms. The electromagnetic coil technique was used to record eye movements [61] . Briefly, a search coil (Skalar BNV, Holland) was inserted below the ocular sclera, and the subject was exposed to two magnetic fields alternating at different frequencies. The demodulation (DNI) of the induced voltage in the coil at these two frequencies then allows simultaneous measurement of horizontal and vertical eye movements. Experimental protocols have been approved by the Marseille Ethical Committee in Neuroscience (approval #A10/01/13, official national registration #71-French Ministry of Research). All procedures complied with the French and European regulations for animal research, as well as the guidelines from the Society for Neuroscience. VSD imaging protocol Experimental controls and online eye position monitoring were performed by a PC running the REX software (NEI-NIH) with the QNX operating system [62] . Optical signals were recorded with a Dalstar camera (512 × 512 pixels, 110 Hz frame rate) driven by the Imager 3001 system (Optical Imaging Ltd.). Both online behavioural control and image acquisition were heartbeat regulated. Heartbeat was detected with a pulse oximeter (Nonin 8600V). The visual stimuli were computed online using VSG2/5 libraries and were displayed on a 22 inch CRT monitor at a resolution of 1,024 × 768 pixels. Refresh rate was set to 100 Hz. Viewing distance was 57 cm. Luminance values were linearized by means of a look-up table. Visual stimuli During a single trial, the monkey had to fixate on a central red dot for 1–2 s. The animal’s gaze was constrained in a window of 2° × 2°. Stimuli were presented during fixation, and a reward (water drop) was given after the trial if the monkey maintained fixation during the acquisition period. We later verified that the s.d. of eye position during stimulation was 0.32° and 0.28° in the horizontal and vertical axes, respectively. Each trial ran for 510–1,100 ms: 100-ms delay, 10–600-ms stimulation period, 400-ms blank period. Stimuli were local Gaussian blobs with a s.d. of 0.5° in space. Stimuli were presented at 0.5° on the left of the vertical meridian and 3.5° below the horizontal, except where noted ( Fig. 4c ). Four different durations were used: 10, 50, 100 ms (monkey WA), and 600 ms (monkey GR). Linear-model denoising method Stacks of images were stored on hard drives for offline analysis. Preprocessing was carried out with Matlab R2009a (The MathWorks) using the Optimization, Statistics and Signal Processing toolboxes. Data were preprocessed using a linear model-based denoising method as described previously [28] . A physically motivated set of basis vectors was designed by characterizing each source of signal and noise in a series of control experiments. For individual trials, the raw signal was decomposed across these basis vectors. Data were denoised by removing the components that are not linked to the evoked response in each individual trial, including physiological artifacts, environmental noise, and dye bleaching. Data were Z -scored via standard methods for further analysis. Temporal filtering Temporal filtering was carried out with an 8 th -order digital Butterworth filter, forward–reverse in time to prevent phase distortion (see MATLAB function filtfilt ). The cutoff frequencies were 5 and 20 Hz, unless otherwise noted. All results were checked with multiple cutoff frequencies to ensure against parametric sensitivity. Phase-latency maps In the analytic signal framework, a real-valued, narrowband time series is transformed into a phasor rotating in the complex plane. After selecting an appropriate temporal point within the oscillation cycle and before the phase crossing threshold (+72.7 ms for all panels in Fig. 4 ), we look for the temporal latency to a given phase crossing (throughout this work, 0/2 π ) at each channel in the unsmoothed, temporally filtered data. Results were checked with several phase crossing values to ensure robustness. Exact times for between-sample 0/2 π phase crossings were calculated by linear interpolation based on the instantaneous frequency of the signal between the two nearest samples. Because the instantaneous frequencies of individual channels may vary across the tested epoch, tracking phase crossing latency (in absolute time) is the most direct option to precisely compare phase offsets. All phase-latency maps are smoothed via a nonparametric, automated algorithm before averaging across trials for purposes of visualization [63] . For further calculations on the phase-latency maps, however, no smoothing is used. Throughout the analysis, several checks were made to ensure the validity of the analytic signal representation. Reconstruction error for this representation was verified to be negligible [64] . Continuity of the phase variable was assessed via the distribution of angular acceleration values , to ensure against the presence of ‘phase slips’, or sudden discontinuities. Phase derivatives and instantaneous frequency The instantaneous frequency of an analytic signal is the time derivative of phase , and is normally calculated by numerical differentiation of the signal instantaneous phase. In this work, all phase derivatives were recast as complex multiplications. Let x n be a discretely sampled real signal, and let be its analytic representation. The product of X n and its complex conjugate at the next sample produces a new complex sequence whose angle is equal to the instantaneous frequency of the original [30] : In this way, we can estimate the signal instantaneous frequency without phase unwrapping. Phase latency correlation with distance With the raw phase latencies calculated, we then find the position of the minimum of the smoothed phase-latency map, and calculate the Euclidean distance of each pixel from this point. We then compute the linear correlation coefficient of phase latency with distance ( ρ d ), as part of the assessment of a significant propagation on the imaging array at the given temporal point. Phase gradient To compute coherent direction maps of the phase gradient, it was necessary to consider only the low spatial frequency components of the signal, by multiplication of the signal at each time slice with a Gaussian in spatial frequency domain (with 0.53 cyc mm −1 s.d. ); however, for the phase gradient magnitude, no spatial smoothing was used. For convenience in measuring signal against the high-frequency spatial noise, we use the reciprocal of this measure (pixel brightness and contour plot, Fig. 6a ), rendering the higher spatial frequencies as short wavevector lengths. Spiking network model The network model considered here is composed of leaky integrate-and-fire (IF) neurons (75% excitatory, 25% inhibitory) with conductance-based synapses. The network is topographically arranged in one dimension, with length L, and wrapped onto the circle, to avoid boundary effects. As in previous work [45] , [65] , the network has local connections defined by a Gaussian spatial profile: where A scales the distribution to the connection probability ( p c ), ℓ ij is the distance between individual neurons, and σ c is the standard deviation (or spatial spread) of the connectivity profile. The axonal conduction delay between two neurons grows linearly with distance: where d syn is the minimum synaptic delay, and ε c is the axonal conduction velocity [6] . For these simulations, we used the PyNN interface [66] to the NEST simulation environment [67] , with a standard IF neuron model and conductance-based alpha-function synaptic inputs ( IF_cond_alpha ). The relevant parameters for the cells and the network are given in Supplementary Table 1 . All other parameters for the model neurons may be found in the PyNN documentation ( http://www.neuralensemble.org/docs/PyNN/standardmodels.html ). To deliver a stimulus to the middle 100 excitatory neurons in the network, we used the Gaussian pulse packet module in NEST ( pulsepacket_generator ), which distributes N sp spikes to each target neuron, following a Gaussian distribution in time, with parameters μ sp and σ sp . As mentioned in the main text, the pulse packet stimulus ignites a wave of subthreshold activity, that is, only 10–20% of spikes in the network occur outside the stimulation zone. To analyse the results of the simulations, we selected six equal, symmetric regions based on the distance from the edge of the stimulation zone, average the V m waveforms over these regions, lowpass filter (4th-order Butterworth, 100 Hz cutoff frequency), and put the resulting waveform into its analytic signal representation. The cross-trial phase distributions were then constructed from the signal phase at the temporal point +115 ms into the simulation. To facilitate comparison between model and experiment, the measured phase values were then rotated by π /2 and multiplied by a complex exponential term to have the same frequency sign as in the experimental data. Note that relative phase values were unchanged by this procedure. Additional checks were performed at each step to ensure the resulting signal is free from discontinuities (for example, the spike reset of the IF neuron), and is well-captured by the final analytic signal representation, so that the comparison between phase variables in the experimental data and the model is well controlled. Finally, additional analysis was performed on the phase distribution of the synaptic conductance variables, which have no such reset discontinuity, to confirm the results of the phase distribution analysis in the model. Circular correlation coefficient To quantify the phase synchronization between neighbouring cortical areas in our VSD data, we computed the pixel-by-pixel circular correlation coefficient [40] , [68] , [69] . For two angular sequences α i and β i of length N with angular means and , the circular correlation coefficient ( ρ cc ) is: To compute the circular correlation coefficient at each time point in these data, we first selected rectangular regions of interest with an equal number of channels. After putting the time courses in each area into their analytic signal representation, we flipped the V2 map vertically and computed the circular correlation coefficient on the phase angles of the aligned pixel pairs in each region. This computation thus estimates the correlation between the spatial pattern of phase in each area. To exclude the regions receiving feedforward input for the thalamocortical input control (light blue dashed line, Fig. 10a ), we selected a region of low-phase latency in the V1 trial-averaged phase-latency map (from +35 to +40 ms), and shuffled the channels within in this region only (15.5% of the V1 ROI). In all cases, image sequences were confirmed to be well registered by manual inspection of both the amplitude and phase maps of the system. Note finally that all means and standard errors of the mean (s.e.m.) were obtained via Fisher z -transform. Analytic signal representation of the gaussian pulse As a control on the spatiotemporal form of the population response in visual cortex, we used a simple model of space timeseparable dynamics, termed ‘Gaussian pulse’ in the text. Again, we write this as a separable function of space and time, where g ( x ) represents a Gaussian profile in space, and h ( t ) is a sinusoidal response time course, with amplitude A , spatial spread σ , and angular frequency ω . We may then take the Hilbert transform of f ( x , t ), and evaluate H [ h ( t )], Now, forming the analytic signal z ( x , t ), which has the form of equation (3) in the main text. Note that an arbitrary phase shift can be added directly into the complex exponential term in equation (22), although this was not written explicitly here. How to cite this article : Muller, L. et al . The stimulus-evoked population response in visual cortex of awake monkey is a propagating wave. Nat. Commun. 5:3675 doi: 10.1038/ncomms4675 (2014).